An experimental test on the probability of extinction of new genetic variants In 1927, J.B.S. Haldane reasoned that the probability of fixation of new beneficial alleles is twice their fitness effect. This result, later generalized by M. Kimura, has since become the cornerstone of modern population genetics. There is no experimental test of Haldane’s insight that new beneficial alleles are lost with high probability. Here we demonstrate that extinction rates decrease with increasing initial numbers of beneficial alleles, as expected, by performing invasion experiments with inbred lines of the nematode Caenorhabditis elegans . We further show that the extinction rates of deleterious alleles are higher than those of beneficial alleles, also as expected. Interestingly, we also find that for these inbred lines, when at intermediate frequencies, the fate of invaders might not result in their ultimate fixation or loss but on their maintenance. Our study confirms the key results from classical population genetics and highlights that the nature of adaptation can be complex. When a new allele appears by mutation or recombination, it will be represented in very low numbers and it can be lost even when it is adaptive. This idea was first formalized by J.B.S. Haldane when he deduced that the probability of fixation of a new beneficial allele is twice its fitness effect [1] . Haldane’s insight became the foundation of modern population genetics [2] , [3] , [4] , [5] and has since been used to understand the limits of adaptation [6] , [7] , [8] , [9] , speciation rates [10] , [11] , [12] and the extent of differentiation between populations [13] , [14] , including those of pathogens and their human hosts [15] , [16] , [17] . Haldane’s result only applies to beneficial alleles and it depends on the invader and resident alleles having independent growth dynamics that will compete in populations characterized by discrete non-overlapping generations and stable sizes [1] , [18] , [19] , [20] , [21] , [22] . His approximation is further conditional on alleles having weak fitness effects and on individuals having successful offspring numbers that follow Poisson distributions. Together, these assumptions allow for genetic drift to be described as a branching process and for the probability of fixation to be calculated from selection coefficients, which in turn can be measured in finite populations as the relative frequency changes of invader and resident alleles [23] . The critical prediction made by Haldane is that, even with a substantial selection advantage, the probability of extinction declines with the number of individuals carrying the invading beneficial allele. There are no explicit experimental tests of this prediction. Results concerning the extinction of beneficial alleles are few [24] , [25] , with the most relevant ones coming from recent experiments where it was shown that the probability of extinction declines with increasing strength of selection [24] . In this latter study, however, extinctions due to genetic drift had to be modelled because the manipulation of the number of invader alleles was not possible. Here we use highly replicated experiments in the hermaphroditic nematode Caenorhabditis elegans to introduce beneficial alleles at precise low numbers in a resident population composed of deleterious alleles to test Haldane’s prediction. The C. elegans model system We started by deriving a collection of inbred lines through self-fertilization of hermaphrodites of a polymorphic population that had been adapted for 140 generations to laboratory conditions. These laboratory conditions involved maintaining stable census population sizes of 10 4 individuals, and effective population sizes of 10 3 , under discrete non-overlapping generations [26] , [27] . In preliminary trials, the derived inbred lines were characterized for embryo to adult survival, with the one showing the lowest values (here referred to as the wild-type line) being chosen as the potentially deleterious surrogate for the resident allele. In parallel, we introgressed a green fluorescent protein (GFP) genetic construct into the lab-adapted population (see Methods ), while maintaining genetic diversity, and then also enforced self-fertilization to derive another collection of inbred lines homozygous for GFP. One of these GFP lines (here referred to as the GFP line) was arbitrarily chosen as the potentially beneficial surrogate for the invader allele. Note that although henceforth we refer to the wild-type and the GFP inbred lines as two different ‘alleles’, these lines differ among them at many loci throughout the genome with each being composed of isogenic diploid individuals. Defining the invader and resident alleles in this manner prevents artifactual positive results due to the GFP introgression. Though GFP expression is fully penetrant and highly visible across larval and adult life-history stages, and is further known to be stably inserted into the genome [28] , difficulties in scoring GFP individuals could lead to inadvertent estimation of low extinction rates (see Methods ). Haldane’s assumption that competing alleles have independent growth dynamics was easily achieved with the number of generations of selfing employed for the inbred line derivation, which makes them nearly isogenic because the average expected heterozygosity across the genome is <0.01% (refs 3 , 27 ) (see Methods ). In line with this, we genotyped the inbred lines at 29 single-nucleotide polymorphisms (SNPs) and found no heterozygosity in them ( Supplementary Data 1 ). Outcrossing among the inbred lines was expected to be of minor consequence because C. elegans hermaphrodites can only cross-fertilize their oocytes when mated with males [29] . Males were initially absent due to the derivation of the inbred lines by selfing, and neither mutation nor selection for outcrossing was expected to increase male frequency for the short duration of the experiments [26] , [30] . Together, these observations imply that segregation and recombination in the two inbred lines would be negligible during the experiments. The inbred lines were thus expected to accurately model haploid, or allelic, growth dynamics that are independent of each other. Beneficial alleles are lost by genetic drift To test for a decrease in extinction rates with the number of beneficial invaders, we performed experiments with two starting frequencies of the GFP allele: either two or five GFP reproductively immature individuals (late L4 larval stage) were introduced into populations with 10 3 wild-type individuals of the same stage. Multiple replicate invasions were seeded and independently propagated for five generations in the same discrete non-overlapping generations experienced by the lab-adapted population during the preceding 140 generations. As total offspring numbers before sampling can reach several tens of thousands ( Supplementary Fig. S1 ), there will be great culling to maintain constant population sizes of N =10 3 , and thus the distributions of successful offspring numbers most likely follow Poisson distributions [18] . The probability of extinction ( P ext ) was measured as the proportion of replicate invasions that failed to show the GFP allele when scored in adult worms, before reproduction, for two consecutive generations (see Methods ). Though extinction of invaders is expected to predominantly occur in the first few generations, genetic drift will nonetheless lead to further loss until tens to hundreds of generations, depending on the initial number of invaders and strength of selection ( Supplementary Fig. S2 ). Note, however, that running the experiments for longer periods at the large population sizes employed would allow mutations to start accumulating [31] , [32] . Results from the two invasion experiments show, as expected, that the P ext was higher when invader alleles started from lower frequencies ( Fig. 1a,b ). In particular, by generation 5, the GFP allele was lost from 37% of the replicates when it started the invasions from two individuals ( n =35, bootstrap 95% confidence interval (CI)=23–51%), but only lost from 12.5% of the replicates when starting from five individuals ( n =56, bootstrap 95% CI=5–21%). To confirm that these results were not biased by an insufficient number of replicates, we next sought to determine if selection on the GFP allele was congruent among the two invasion experiments. 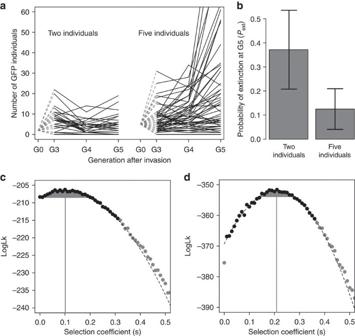Figure 1: Extinction decreases with number of invading alleles. (a) The dynamics of invasions. Observed number of GFP individuals, when two or five individuals initially invade a population withN=103wild-type individuals. Thirty-five replicates were used in the experiments starting with two GFP individuals, whereas 56 replicates were followed in the invasions with five GFP individuals. (b) Observed probability of extinction at G5 with 2 s.d. of 1,000 bootstrap replicates is shown as the error bars. (c,d) Selection coefficient estimates. For the two-individual (c) and five-individual (d) GFP invasion experiments, the likelihood values of selective coefficients (s) for the observed GFP allele counts at G3, G4 and G5 are presented. These were obtained by simulations of 108invasions. In the region close to the initial ML estimate, defined as ML-10log10(black circles), an extra set of 9 × 108simulations were performed. A quadratic function was then fitted to this interval (dashed line) to obtain the final ML estimate ofs(grey line) with −2log10confidence limits (grey area). Figure 1: Extinction decreases with number of invading alleles. ( a ) The dynamics of invasions. Observed number of GFP individuals, when two or five individuals initially invade a population with N =10 3 wild-type individuals. Thirty-five replicates were used in the experiments starting with two GFP individuals, whereas 56 replicates were followed in the invasions with five GFP individuals. ( b ) Observed probability of extinction at G5 with 2 s.d. of 1,000 bootstrap replicates is shown as the error bars. ( c , d ) Selection coefficient estimates. For the two-individual ( c ) and five-individual ( d ) GFP invasion experiments, the likelihood values of selective coefficients ( s ) for the observed GFP allele counts at G3, G4 and G5 are presented. These were obtained by simulations of 10 8 invasions. In the region close to the initial ML estimate, defined as ML-10log 10 (black circles), an extra set of 9 × 10 8 simulations were performed. A quadratic function was then fitted to this interval (dashed line) to obtain the final ML estimate of s (grey line) with −2log 10 confidence limits (grey area). Full size image For this, we numerically simulated the expected change in GFP allele frequency during the invasion experiments as a function of its relative fitness, while accounting for the total number of individuals and the life cycle of the populations. Specifically, the relative growth rates of GFP and wild-type alleles were modelled as 1+ s and 1, respectively, with s being defined as a selection coefficient [3] . We estimate selection not by an analytical approach, which determines the ultimate probability of fixation for weak or strong selection, but by exact Monte–Carlo simulations (see Methods ). Maximum likelihood (ML) analyses of the allele counts done during the last three generations of the experiments confirmed our initial suspicion that the GFP inbred line was fitter than the wild-type inbred line, regardless of initial numbers ( Fig. 1c,d ). The estimated selection coefficient for the GFP allele is consistent between the two experiments; as the estimates have overlapping confidence limits ranging from s =0.14 to s =0.20. Among experiments, the mean selection coefficient of the GFP allele was of 0.16. Together, the probability of extinction measured at generation 5 and the selection coefficients estimated demonstrate that genetic drift was responsible for the loss of beneficial alleles during the first generations after their invasion. Deleterious alleles temporally evade genetic drift In contrast to the fate of beneficial invader alleles, deleterious alleles can reach high frequencies by genetic drift when N e s <1 (refs 5 , 20 , 21 , 22 ). Although in our case Ns >10, theory nevertheless predicts that the extinction rates of a rare deleterious allele should be higher than that of an invading beneficial allele of equivalent absolute fitness. We next tested this prediction by asking whether or not inverting the direction of the invasions would lead to higher P ext , and if so the selection coefficient would be of similar magnitude but negative in sign. For this second set of invasion experiments, five individuals from the wild-type inbred line were introduced into a population with 10 3 GFP individuals. Results show that after five generations the wild-type allele had been lost in 56% of the replicates ( Fig. 2a ). This was a proportion, which, as expected, was much higher than that observed when the five GFP individuals invaded the wild-type population (from Fig. 1b , 12.5%). Furthermore, the median selection coefficient that best explained the P ext of the (deleterious) wild-type allele was of −0.138 ( Fig. 2a ), which in magnitude, and also as expected, closely matched the selective coefficient of the GFP allele found in the first set of invasion experiments (from Fig. 1c,d ; mean s =0.16). 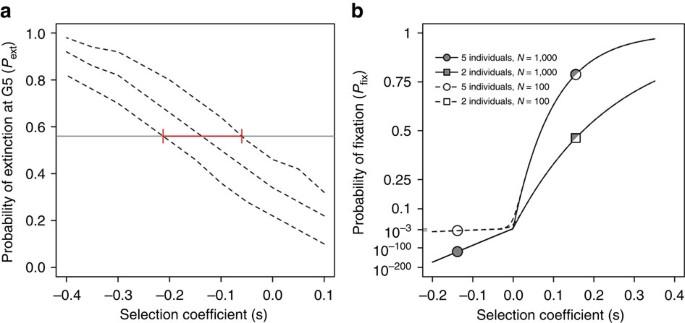Figure 2: Probability of extinction and fixation. (a) Observed probability of extinction at G5 when five wild-type individuals invade a population with 103GFP individuals (grey line). Fifty replicate invasions were followed. The interquantile range of the median probability of extinction (dashed lines) was obtained by numerical simulations of the invasion experiment with selection coefficient between −0.4 and 0.1. The median selection coefficient that best reflects the observed number of line losses is ofs=−0.138, with the red error bar indicating the expected interquantile range (n=103simulations). (b) Expected probability of fixation of invader alleles, using M. Kimura diffusion process approximation, obtained for the selective coefficients estimated from the three invasion experiments performed (symbols). Lines indicate the probability of fixation withN=103or 102and constants=0.16 or −0.138 (for probability of fixation with frequency-dependent selection, seeFig. 4). With strong selection on beneficial invaders, the probability of fixation is the same for the two population sizes (half-filled symbols). For strong selection, the approximation, wherenis the number of beneficial invaders, is indistinguishable from Kimura’s approach employed here33. The probability of fixation scale is truncated for clarity. Figure 2: Probability of extinction and fixation. ( a ) Observed probability of extinction at G5 when five wild-type individuals invade a population with 10 3 GFP individuals (grey line). Fifty replicate invasions were followed. The interquantile range of the median probability of extinction (dashed lines) was obtained by numerical simulations of the invasion experiment with selection coefficient between −0.4 and 0.1. The median selection coefficient that best reflects the observed number of line losses is of s =−0.138, with the red error bar indicating the expected interquantile range ( n =10 3 simulations). ( b ) Expected probability of fixation of invader alleles, using M. Kimura diffusion process approximation, obtained for the selective coefficients estimated from the three invasion experiments performed (symbols). Lines indicate the probability of fixation with N =10 3 or 10 2 and constant s =0.16 or −0.138 (for probability of fixation with frequency-dependent selection, see Fig. 4 ). With strong selection on beneficial invaders, the probability of fixation is the same for the two population sizes (half-filled symbols). For strong selection, the approximation , where n is the number of beneficial invaders, is indistinguishable from Kimura’s approach employed here [33] . The probability of fixation scale is truncated for clarity. Full size image Having shown that genetic drift has an impact on the establishment of beneficial and deleterious alleles, we can ask what are their expected probabilities of fixation ( P fix ). For this, we turned to M. Kimura’s diffusion approach that generalizes Haldane’s result to both beneficial and deleterious alleles [20] , [21] : , where p is the initial frequency of the invader allele, and N e is the effective size of the population. With N e =10 3 , the expected P fix of a beneficial allele would be 0.46 or 0.79 when invading a population with two or five individuals, respectively ( Fig. 2b ). If the invader allele is deleterious, fixation is impossible with just five individuals and N e =10 3 . If during the invasion experiments sizes were of N e =10 2 or lower, which reflects typical situations when the effective population sizes are smaller than the census population sizes [9] , [27] , the P fix of a deleterious allele would increase and likely become significant. For the calculations of P fix , the assumption of weak selection is violated because high selection coefficients were found. For beneficial alleles, when N e s>> 1, Kimura’s expression shown above simplifies to , with n being the number of invaders, which predicts no dependence on population sizes (as also shown in Fig. 2b ). Yet, even with strong positive selection, the P fix is expected to be different when two or five individuals invade a resident population. Furthermore, it has been previously shown that, with not very high selection coefficients, relatively small discrepancies in P fix between Kimura’s diffusion approach and simulations of genetic drift under several explicit demographic scenarios are expected [33] , [34] . Kimura’s approach, even if originally devised for weak selection, should thus remain a good approximation of the ultimate P fix of an invader allele, whether it is beneficial or deleterious, in the range of selection coefficients explored here. Frequency-dependent selection might maintain polymorphism In Haldane’s result, the probability of fixation of rare beneficial alleles is conditional only on their survival during the initial stages of the invasion, where extinction by genetic drift is common. It is possible, however, that with frequency dependence, successful invasions of beneficial alleles do not ultimately result in their fixation. Our final experiments were done to illustrate this possibility by competing of the same wild-type and GFP inbred lines, but now at starting intermediate frequencies. As the invasion experiments above, these intermediate-frequency experiments were run for multiple generations, and scoring of the GFP was done at the adult life stage. Setup was, however, done at the first larval stage (L1 stage) as it would have been extremely difficult to separately handpick thousands of individuals and have adequate replication. Again as in the invasion experiments, the demographic conditions of discrete non-overlapping generations at N =10 3 were followed. This time, we used the deterministic expectations of GFP allele frequency change over generations to estimate selection [3] , [19] (see Methods ). Strikingly, when GFP and wild-type inbred lines were competed at approximately equal proportions, a significant decrease in GFP alleles was observed ( Fig. 3a ). At intermediate frequencies, the GFP allele was therefore found to be deleterious (mean s =−0.12), contrary to the beneficial fitness effect that we found when it invaded populations from low frequencies. During the first generation of this intermediate-frequency experiment, we also scored the GFP allele frequency at the L1 larval stage. When comparing the selection coefficients estimated from a single generation of competition at the L1 and the adult stage, no differences were detected ( Fig. 3b ). Independently of the protocol employed therefore, whether it is single or multi-generational or whether scoring is done at the L1 or at the adult stage, the GFP allele was consistently deleterious when at intermediate frequencies. 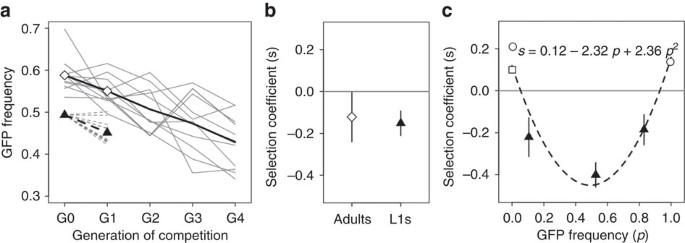Figure 3: Frequency-dependent selection. (a) The GFP allele is deleterious. Intermediate-frequency competitions between the GFP and the wild-type inbred lines show that the GFP allele declines in frequency. GFP allele frequency changes are shown for 11 replicate competitions (grey lines). The mean GFP frequency in adults through time is shown as a black line. The mean selection coefficient estimated from multiple generations, at the adult stage, iss=−0.12±0.03 s.d. (seeMethods). The frequency declines in GFP allele observed over one generation both at the L1 stage (dashed grey lines) and at the adult stage (solid grey lines) are shown. (b) Estimated selection coefficients at adult and L1 stages for GFP allele frequency changes in a single generation, froma(symbols), show no effect of life-history stage (Welch’st-test,t14.7=−0.45,P=0.66). Error bars indicate 2 s.e.m. among the 10 replicates at each stage. (c) The form of frequency-dependent selection. Estimated selection coefficients from one-generation competition experiments at several intermediate initial GFP frequencies are shown as triangles. Measurements were done at the L1 stage. Error bars indicate 2 s.e.m. among the 10 replicates for each starting frequency. Selection coefficient estimates from the invasion experiments with two (square) or five (circle) starting GFP individuals are also shown as empty symbols (from the data inFigs 1cand2a). Note that the selection coefficient estimated from the invasion experiment where the GFP allele was at an initial proportion of 0.995 is the absolute selection coefficient of the wild-type invader allele. Frequency-dependent selection is illustrated by a quadratic regression on all data points (R2=0.91; inset). Neutrality is indicated as a grey line. Figure 3: Frequency-dependent selection. ( a ) The GFP allele is deleterious. Intermediate-frequency competitions between the GFP and the wild-type inbred lines show that the GFP allele declines in frequency. GFP allele frequency changes are shown for 11 replicate competitions (grey lines). The mean GFP frequency in adults through time is shown as a black line. The mean selection coefficient estimated from multiple generations, at the adult stage, is s =−0.12±0.03 s.d. (see Methods ). The frequency declines in GFP allele observed over one generation both at the L1 stage (dashed grey lines) and at the adult stage (solid grey lines) are shown. ( b ) Estimated selection coefficients at adult and L1 stages for GFP allele frequency changes in a single generation, from a (symbols), show no effect of life-history stage (Welch’s t -test, t 14.7 =−0.45, P =0.66). Error bars indicate 2 s.e.m. among the 10 replicates at each stage. ( c ) The form of frequency-dependent selection. Estimated selection coefficients from one-generation competition experiments at several intermediate initial GFP frequencies are shown as triangles. Measurements were done at the L1 stage. Error bars indicate 2 s.e.m. among the 10 replicates for each starting frequency. Selection coefficient estimates from the invasion experiments with two (square) or five (circle) starting GFP individuals are also shown as empty symbols (from the data in Figs 1c and 2a ). Note that the selection coefficient estimated from the invasion experiment where the GFP allele was at an initial proportion of 0.995 is the absolute selection coefficient of the wild-type invader allele. Frequency-dependent selection is illustrated by a quadratic regression on all data points ( R 2 =0.91; inset). Neutrality is indicated as a grey line. Full size image To further support the change in the sign of selection, we repeated the competitions but now starting from three different intermediate GFP proportions (see Methods ): 0.15, 0.5 and 0.85. These experiments were run for a single generation, and the GFP allele frequency was measured at the L1 larval stage, again to have adequate replication. Results show that the GFP allele continued to be deleterious for these different intermediate frequencies ( Fig. 3c , mean s between −0.18 and −0.40). When the selection coefficients estimated from the latter experiments and from the invasion experiments are plotted together with their corresponding starting GFP frequencies, a non-linear function clearly emerges ( Fig. 3c ). Positive selection coefficients at the extreme frequencies employed in the invasion experiments demonstrate that individuals carrying the GFP allele can escape loss when rare or, alternatively, resist the invasion of the wild-type allele. When between 5 and 93%, however, selection will be against the GFP allele. In other words, there was frequency-dependent selection among the two inbred lines. It is possible that underlying frequency-dependent selection are differences in the reproductive behaviour of the two inbred lines, as they seem to differ in embryo laying and embryo retention rates, as well as in successfully propagating themselves in our specific culture protocol ( Supplementary Figs S1 and S3–S5 ). Interactions among fitness components are nevertheless complex, and only a comprehensive characterization of several life-history traits would allow a full understanding of the possible mechanisms underlying the observed frequency dependence, an endeavour that is beyond the scope of the present study. We finish by showing that the successful invasion of beneficial alleles in a population might not necessarily lead to their ultimate fixation. From the fitness function of Fig. 3c , it is apparent that there are two equilibrium frequencies but only one of them is stable, at around 5%. Taking as an example the invasion experiments that were seeded with five GFP individuals, frequency-dependent selection or frequency-independent selection would initially have similar consequences to the extinction of beneficial invaders because they would be relatively rare ( Fig. 4a ). After 100 generations or so, however, and with frequency-independent selection, most of the populations where extinction did not occur would be fixed for the beneficial invader allele. In contrast, with frequency-dependent selection, polymorphism would be maintained at the stable equilibrium frequency. One of the expected outcomes of evolution under frequency-dependent selection is thus the maintenance of polymorphism for longer periods than under frequency-independent selection ( Fig. 4b,c ). If, however, the stable equilibrium frequency is of sufficiently low value, genetic drift can lead to higher extinction rates than those expected with frequency-independent selection ( Fig. 4c , dashed lines). Higher extinction of new beneficial alleles is therefore expected to be important for populations with small sizes, as in them genetic drift is more pronounced. 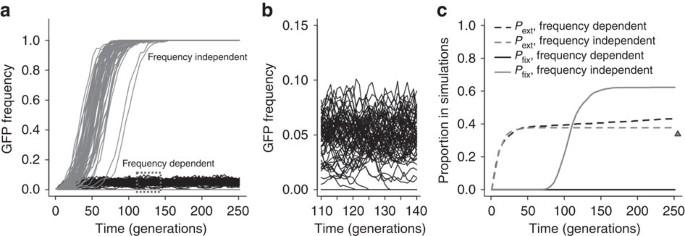Figure 4: Selection may maintain diversity and increase extinction. (a) GFP allele frequency dynamics in simulated populations when starting with five GFP invaders. Simulations were run under frequency-dependent (black) or frequency-independent selection (grey), wheres=0.12–2.32 p+2.36p2ors=0.108 (assumed constant and calculated withP=0.005), respectively (fromFig. 3c). The stable polymorphic equilibrium is rapidly reached at around 5% under frequency-dependent selection, while most fixations occurred by generation 100 under frequency-independent selection. (b) Enlargement of the dashed box inafor frequency-dependent selection. Several replicate populations face extinction even when their sizes were simulated withN=103. (c) Expected probabilities of extinction and fixation estimated from the 1,000 simulated populations ofaandb, under frequency-dependent selection or frequency-independent selection (black or grey lines). Frequency-dependent selection can increase extinctions when compared with frequency-independent selection after generation 50 (dashed lines). The triangle indicates the ultimate probability of extinction (infinite time) when using the approximationPext=e−2sfor frequency independence with large selection coefficients33. Figure 4: Selection may maintain diversity and increase extinction. ( a ) GFP allele frequency dynamics in simulated populations when starting with five GFP invaders. Simulations were run under frequency-dependent (black) or frequency-independent selection (grey), where s =0.12–2.32 p+2.36 p 2 or s =0.108 (assumed constant and calculated with P =0.005), respectively (from Fig. 3c ). The stable polymorphic equilibrium is rapidly reached at around 5% under frequency-dependent selection, while most fixations occurred by generation 100 under frequency-independent selection. ( b ) Enlargement of the dashed box in a for frequency-dependent selection. Several replicate populations face extinction even when their sizes were simulated with N =10 3 . ( c ) Expected probabilities of extinction and fixation estimated from the 1,000 simulated populations of a and b , under frequency-dependent selection or frequency-independent selection (black or grey lines). Frequency-dependent selection can increase extinctions when compared with frequency-independent selection after generation 50 (dashed lines). The triangle indicates the ultimate probability of extinction (infinite time) when using the approximation P ext = e −2 s for frequency independence with large selection coefficients [33] . Full size image We have shown that even beneficial alleles with strong fitness effects can be lost by genetic drift, if they have not reached a high enough frequency for their dynamics to become deterministic [1] , [18] , [19] . Deleterious alleles on the other hand can escape genetic drift and be maintained at relatively high frequencies, particularly in small populations, at least until selection efficiently purges them [20] , [21] , [22] . Together, the invasion experiments clearly confirm classical theory in population genetics [2] , [3] , [4] , [5] . As also shown, however, once beneficial alleles are established in a population, they might not speed to fixation, but be maintained, because at intermediate frequencies their adaptive values can change in sign. Though the generality of frequency-dependent selection remains to be shown, our observations from the intermediate-frequency experiments in these strains might be relevant for interpreting variation in natural populations that are genetically structured by variation in ploidy levels [35] , [36] , assortative mating and inbreeding among relatives [14] , [37] , population subdivision [38] , [39] or repeated hybridization [40] , [41] . In all of them, frequency-dependent selection might be common, which together with genetic drift can hinder adaptation to novel environments. In conclusion, classical theory in population genetics is confirmed, but natural selection might not be of invariable magnitude and sign. Our findings thus set the stage for the development of more general theoretical models explaining the fate of new alleles across long evolutionary timescales [22] , [42] , [43] , [44] . Inbred lines The wild-type inbred line (EEV1401) was derived by 12 consecutive generations of self-fertilization of hermaphrodites coming from a polymorphic lab-adapted population (A6 140 ). Twenty wild-type inbred lines were derived by the expansion of the last generation of self-fertilization to high sample sizes (>10 3 ) during two generations. M9 solutions containing arrested L1-staged individuals were mixed in equal proportions to a solution of 1 M NaCl, 1 M KH 2 PO 4 , glycerine and 1 M MgSO 4 , with stocks being then frozen at −80 o C (ref. 45 ). The lab-adapted population had been maintained for 140 generations under discrete non-overlapping generations at constant population census sizes of N =10 4 (refs 26 , 27 ). As determined at SNPs covering 1/3 of the genome, the effective population sizes were of N e =10 3 until generation 100 of experimental evolution [26] , [27] . To derive an inbred line that would allow easy scoring during the experiments reported here, the genome-integrated transgenic array ccls4251(myo-3::GFP) [28] , from strain PD4251, was first introgressed into A6 140 . The transgenic array is stable and expressed in muscle cells of all larval and adult stages [28] . Outcrossing of PD4251 males with A6 140 hermaphrodites was followed by three consecutive generations of self-fertilization to obtain separate GFP F2 families. As the GFP is dominant, only F2 individuals coming from families where all relatives expressed it were kept for the next introgression cycle. Five of these introgression cycles were done, each starting with the mating of GFP homozygous F2 hermaphrodites to an excess of males from A6 140 . Five to ten families were employed at each introgression cycle to ensure maintenance of diversity. Once this A6 140 GFP population was constructed, 10 consecutive generations of self-fertilization in hermaphrodites were done to derive three inbred GFP lines. One of these was arbitrarily chosen for the experiments (EEV1402). Inbred line genetic diversity The extent of heterozygosity within each inbred line was determined by genotyping 29 SNPs in pools of 20–30 individuals ( Supplementary Data 1 ). These SNPs are located in chromosome IV and are not under high linkage disequilibrium in the A6 140 population (mean r 2 =0.03 (ref. 27 )). Genomic DNA form was prepared with the ZyGEM prepGEM Insect kit following the manufacturer’s protocol. Genotypes were mass determined with allele-specific extension reactions on oligonucleotides generated from PCR-amplified genomic DNA using the iPlex Sequenom MALDI-TOF platform [27] , [46] . Expected heterozygosities upon inbreeding were obtained by: H t =1−[(1/2) t H 0 ] (ref. 3 ), with H 0 =0.24 being the average heterozygosity of A6 140 measured at 334 SNPs, H the Hardy–Weinberg proportions and t the number of generations of self-fertilization. Culturing of populations Inbred lines were revived for each set of experiments from −80 o C stocks and expanded for two generations under a common environment before setup. All replicates were separately passaged under discrete 4-day non-overlapping life cycles at constant sizes of 10 3 individuals. Developmental synchronization occurred at the first larval stage (L1), after which seeding was done to 9 cm petri plates with NGM-lite agar (US Biological), carrying a fully confluent lawn of Escherichia coli (HT115 strain). After 72±2 h of growth under constant temperature (20° C) and relative humidity (80%), worms were removed from the plates, subjected to a 1 M KOH: 5% NaOCl solution for 5min and repeatedly washed in M9 buffer. Only the embryos that were laid in the plates and transferred, together with those that burst out of the hermaphrodite body, survived this procedure ( Supplementary Fig. S3 ). After 24±2 h, L1s were collected to seed the following generation. Densities were estimated by scoring the number of L1s in five 5 μl samples ( Supplementary Fig. S6 ). Invasion experiments For the experiments where the GFP line was the invader, 35 petri dishes were set up, each with two immature late L4 individuals (L4s; 48±2 h after L1 seeding), whereas 56 petri dishes were set up with five individuals, in a resident population of 10 3 wild-type individuals of similar developmental stage. All these were concurrently passaged for five generations. Setup was thus done before reproduction (G0). At G1 and G2, plates were only scored for presence/absence of GFP individuals, and from G3–G5 all individuals were scored. Loss of GFP was only considered if it could be confirmed in two consecutive generations. For the experiments where the wild-type line was the invader, 50 petri dishes were set up with five individuals. These were done at a different time and thus involved another revival of the lines from the −80 o C stocks. In these experiments, only a sample of 300 individuals were scored from G1 to G5. GFP loss was declared if the wild-type individuals failed to be detected for three consecutive generations. The probability of extinction measured at G5 had thus to include observations from extra G6 and G7. Invaders were scored at the adult stage before passage with a stereoscope equipped with a mercury lamp and GFP filters at × 15 magnification. For the exact counts of GFP individuals, see Supplementary Tables S1 and S2 . Selection in invasion experiments In the experiments with GFP individuals as invaders, selection coefficients ( s ) were obtained by ML using Monte–Carlo numerical simulations. Each simulation started with the initial invader frequencies at fixed 2 × 10 −3 or 5 × 10 −3 that were sampled following: where t is generation [3] , [19] . Equation (1) thus formulates the expected frequency change of a GFP allele with growth rate 1 +s relative to a wild-type allele of growth rate 1. A random number of GFP alleles were sampled for four generations, following a binomial distribution with p t+1 as the probability of success and 10 3 as the sample size. 10 8 replicate simulations were done for each invasion experiment and for each of 101 selection coefficients defined in a grid of points between 0 and 1. At G3, G4 and G5, the empirical likelihood estimates were obtained by comparison of simulated and observed GFP individual counts. In the range where likelihood values were higher than the ML minus 10 log-likelihoods, 9 × 10 8 extra replicate simulations were performed. A quadratic function was then fitted to these intervals to obtain the ML estimate minus 2 log-likelihoods for CIs. In this last step, experimental data that were not observed in at least 50 simulations, for any given s , were removed to reduce noise. In the experiments with wild-type individuals as invaders, the interval of s values compatible with the number of observed line losses at G5 was obtained in a similar manner. Replicate simulations of 10 3 were done for selection coefficients defined in a grid of points between −0.4 and 0.1. One extra step in the algorithm relative to that above was introduced after experimental passage to reflect the sampling of 300 individuals for scoring. As for the experimental data, extinction was declared when the invader was not observed for three consecutive generations until G7. The proportion of replicates where extinctions occurred by G5 were recorded as the median value and the interquantile range, because the simulated data were not normal. Linear interpolation was used to find the best estimate of s and its error range. All computations were done using R [47] . Intermediate-frequency experiments Inbred lines were revived from −80 o C stocks and expanded for two generations under common environmental conditions. On the third generation, L1-staged GFP individuals were mixed with L1-staged wild-type individuals at a proportion of 0.5. The GFP frequencies observed in the adults of that generation constituted the starting frequencies for the estimation of selection coefficients in the adult stage. Eleven replicate competitions were then passaged for four generations in the same conditions employed for the invasion experiments. The mean number of adults scored per replicate and generation was of 767 and not less than 414. Estimates of GFP frequency changes were also obtained from L1-stage individuals for the set-up frequencies and after one generation (see below) to compare estimates between L1 and adult stages. For the characterization of frequency dependence, GFP and wild-type L1s were mixed at three different starting proportions: 0.15, 0.50 and 0.85. These intermediate-frequency experiments were conducted at a different time and thus involved yet another revival of the inbred lines from the −80 o C stocks. For each starting frequency, 10 replicate competitions were done by seeding 10 3 individuals. GFP scoring was done in the following generation at the L1 larval stage, by placing 5 μl of the M9 buffer containing L1s on glass slide and photographing them at 2 pixel μm −1 resolution under a microscope equipped with a GFP filter. The mean number of L1s scored per replicate competition was of 1,159 and not less than 762. Allele frequency estimates were similarly obtained for the starting mixes to estimate sampling error ( Supplementary Fig. S6 ). Selection in the intermediate-frequency experiments For the multiple generation experiment where adults were scored, selection coefficients were obtained by solving equation (1) shown above, given the observed GFP allele frequencies. A mean selection coefficient ( ŝ ) was obtained from the intercept of a mixed model, where replicate competitions where used as a random factor. The calculation of different selection estimates separately at the several generations indicated congruency among them, and hence time was not included in the model. The resulting selection coefficient is thus the mean s obtained from the different replicate competitions. Note that the most common estimation method for s , using the log ratio of allele frequencies that changes with time [2] , [48] , would give estimates close to those reported in the main text ( s =−0.16±0.03 s.e.m. with the log ratio method, compared with s =−0.12±0.03 s.e.m. by solving equation (1)). As equation (1) was used in the Monte–Carlo simulations for estimation of selection in the invasion experiments, we continued to use it for the estimation of selection in the intermediate-frequency experiments. Simulations of frequency-dependent selection Monte–Carlo simulations followed the same algorithm as in the invasion simulations with starting GFP proportions of 0.005. At each generation, s was evaluated (from equation (1)) according to the fitness function of Fig. 3c , to model frequency dependence, or by fixing s when at P =0.005 in the same fitness function, to model frequency independence. One thousand replicates in each selection scenario were obtained. P ext and P fix were calculated from the number of replicates where the invader allele was lost or fixed, respectively. How to cite this article: Chelo, I. M. et al . An experimental test on the probability of extinction of new genetic variants. Nat. Commun. 4:2417 doi: 10.1038/ncomms3417 (2013).